Defect-induced supersolidity with soft-core bosons More than 40 years ago, Andreev, Lifshitz and Chester suggested the possible existence of a peculiar solid phase of matter, the microscopic constituents of which can flow superfluidly without resistance due to the formation of zero-point defects in the ground state of self-assembled crystals. Yet, a physical system where this mechanism is unambiguously established remains to be found, both experimentally and theoretically. Here we investigate the zero-temperature phase diagram of two-dimensional bosons with finite-range soft-core interactions. For low particle densities, the system is shown to feature a solid phase in which zero-point vacancies emerge spontaneously and give rise to superfluid flow of particles through the crystal. This provides the first example of defect-induced, continuous-space supersolidity consistent with the Andreev–Lifshitz–Chester scenario. Spontaneous symmetry breaking is a focal principle of condensed matter physics, yet simultaneous breaking of fundamentally different symmetries represents a rare phenomenon. A prime example is the so-called supersolid phase [1] , which displays both crystalline and superfluid properties, that is, the simultaneous breaking of continuous translational and global gauge symmetry. The first mentioning of such a state goes back to Gross [2] , who predicted the possibility of a density-modulated superfluid phase of weakly interacting Bosons described by a classical field. Later, Andreev and Lifshitz [3] , and Chester (ALC) [4] conjectured a microscopic mechanism for strongly interacting systems, based on two key assumptions: first, that the ground state of a bosonic crystal contains defects such as vacancies and interstitials and, second, that these defects can delocalize, thereby, giving rise to superfluidity. However, the physical realizability of this scenario has since remained under active debate [5] . In 2004, torsional oscillator experiments [6] , [7] provided first suggestive evidence for superfluidity in solid 4 He through a rapid drop of the resonant oscillation period below a critical temperature, viewed indicative for superfluid decoupling of a fraction of the He crystal. This finding has sparked a host of new experimental activity [8] , [9] , [10] , [11] , [12] , [13] , [14] , [15] , [16] , [17] , [18] that, however, challenged the original interpretation and pointed out several artefacts causing a non-supersolid origin of the observations. Theoretical work has established that crystal incommensurability is a necessary condition for superfluidity [19] and that zero-point defects in ground-state solid He are prevented by a large activation energy [20] , [21] . In addition, Boninsegni et al. [21] Rota and Boronat [22] , Ma et al. [23] , and Lechner and Dellago [24] have shown that point-like defects experience an effective attraction that results in defect-clustering and phase separation, ruling out the possibility of defect-induced supersolidity [21] as in the ALC scenario. Several experiments [11] , [14] , [15] , [16] have shown that the original observations were caused by shear modulus stiffening of bulk solid He, and later found no signature of superfluidity on avoiding this effect [25] . As a result, there now seems to be consistent experimental and theoretical evidence for the absence of the long-sought supersolid phase in He. The mere existence of continuous-space supersolidity induced by zero-point defects thus remains an open question. In this Article, we show that bosonic particles interacting via soft-core potentials (see Fig. 1 ) provide a prototype system for addressing this question. Using exact numerical techniques, we determine the underlying zero-temperature phase diagram, which reveals the emergence of defect-induced supersolidity in the vicinity of commensurate solid phases, as conjectured by ALC [3] , [4] . 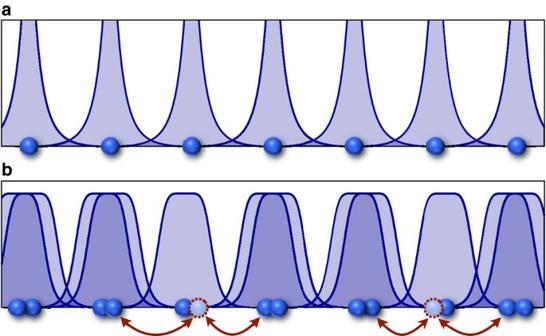Figure 1: Crystallization due to singular and soft-core interactions. (a) For singular potentials with pure power-law repulsion, indicated by the blue areas, particles assemble into a commensurate and insulating solid. (b) On removing the singularity, particles can cluster and, under proper conditions, form an incommensurate crystal with more particles than lattice sites. Defect delocalization due to inter-site tunnelling can then promote a finite superfluid response of the self-assembled crystalline ground state. Figure 1: Crystallization due to singular and soft-core interactions. ( a ) For singular potentials with pure power-law repulsion, indicated by the blue areas, particles assemble into a commensurate and insulating solid. ( b ) On removing the singularity, particles can cluster and, under proper conditions, form an incommensurate crystal with more particles than lattice sites. Defect delocalization due to inter-site tunnelling can then promote a finite superfluid response of the self-assembled crystalline ground state. Full size image Supersolidity with soft-core bosons We consider a two-dimensional ensemble of N bosons with density ρ , interacting via a pair potential of the type This interaction approaches a constant value V 0 / as the inter-particle distance, r , decreases below the soft-core distance R c and drops to zero for r > R c . The limiting case γ →∞ yields the soft-disc model [26] , while γ =3 and γ =6 correspond to soft-core dipole–dipole [27] and van der Waals [28] interactions that can be realized with ultracold atoms [28] , [29] or polar molecules [30] , [31] . Here we focus on the latter case ( γ =6) for which the Hamiltonian reads where the units of length and energy are R c and ħ 2 / m , respectively, and m denotes the particle mass. In these units, the zero-temperature physics is controlled by the dimensionless interaction strength U = mV 0 /( ħ 2 ) and the dimensionless density ρ . Particles with soft-core interactions have been studied previously in the field of soft condensed matter physics [32] , [33] , [34] in the classical high-temperature regime. One of the main findings has been that pair potentials with a negative Fourier component [32] favour the formation of particle clusters, which in turn can crystallize to form a so-called cluster crystal. In the quantum domain, theoretical work has so far focused on the regime of weak interactions and high particle densities [27] , [28] , [35] , [36] , [37] , [38] , which was shown to be well described by mean-field calculations [39] , [40] . In this limit, one finds strongly modulated superfluid states [2] , [26] , [27] with broken translational symmetry in the form of a density wave. In the following, we investigate the strong coupling domain where correlations and quantum fluctuations are expected to become important. We employ path-integral Monte Carlo simulations to determine the ground-state properties of the Hamiltonian equation (2) (see Methods section). The obtained phase diagram, shown in Fig. 2 , reveals a rich spectrum of phases with varying interaction strength and density. 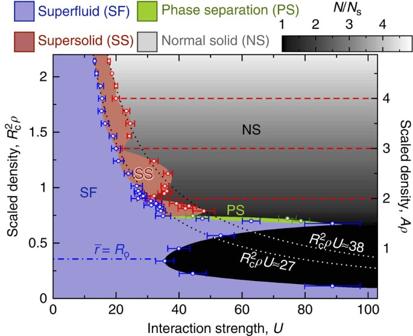Figure 2: Zero-temperature phase diagram of two-dimensional soft-core bosons. The phase diagram displays the emergence of superfluid (SF) and different solid (NS) and supersolid (SS) phases for varying interaction strengthUand densityρ. The density on the leftyaxis has been scaled by the soft-core radiusRc. The right axis gives the density in units of the inverse area,A=(1.6Rc)2/2, of the unit cell of the high-density solid phase, corresponding to the lattice site occupationN/Nsfor a given number of particles and lattice sites,NandNs, respectively. ForAρ≳1.5, the grey region labelled as NS corresponds to a cluster crystal withN/Ns>1, as indicated by the grey scale. Supersolid phases with different occupation numbers are found between two hyperbolas, defined byρU=const. (dotted lines). At high densities (Aρ≳3.5) they can be understood in terms of density-modulated superfluids. In contrast, superfluidity within the low-density supersolid lobes emerges from delocalized zero-point defects according to the ALC scenario. The horizontal error bars represent statistical uncertainties and uncertainties due to the finite stepping ofU. Figure 2: Zero-temperature phase diagram of two-dimensional soft-core bosons. The phase diagram displays the emergence of superfluid (SF) and different solid (NS) and supersolid (SS) phases for varying interaction strength U and density ρ . The density on the left y axis has been scaled by the soft-core radius R c . The right axis gives the density in units of the inverse area, A = (1.6 R c ) 2 /2, of the unit cell of the high-density solid phase, corresponding to the lattice site occupation N / N s for a given number of particles and lattice sites, N and N s , respectively. For Aρ ≳ 1.5, the grey region labelled as NS corresponds to a cluster crystal with N / N s >1, as indicated by the grey scale. Supersolid phases with different occupation numbers are found between two hyperbolas, defined by ρU =const. (dotted lines). At high densities ( Aρ ≳ 3.5) they can be understood in terms of density-modulated superfluids. In contrast, superfluidity within the low-density supersolid lobes emerges from delocalized zero-point defects according to the ALC scenario. The horizontal error bars represent statistical uncertainties and uncertainties due to the finite stepping of U . Full size image Small particle densities At small densities ρ ≲ 0.5, we find two phases: a superfluid and an insulating triangular crystal composed of singly occupied sites, that is, where the number of lattice sites, N s , equals the particle number N . The observed lobe structure of this crystalline region is readily understood by noticing that at very low densities, that is, large inter-particle distances > R c , the physics is dominated by the long-range tail of the interaction potential, V ~1/ r 6 . For a fixed interaction strength U ≳ 35, we thus find a first-order liquid–solid quantum phase transition with increasing Aρ , consistent with previous work on bosons with power-law interactions [30] , [41] , [42] , [43] . In particular, the location of the liquid–solid phase transition for very low densities coincides with that for pure van der Waals interactions. With increasing density, however, the average inter-particle spacing, , approaches the soft-core radius R c and drops to values for which equation (1) strongly deviates from pure ~1/ r 6 interactions and levels off below the turning point R o =(5/7) 1/6 R c . As a result of the decreasing repulsive inter-particle forces, the crystal melts again for increasing densities. As indicated in Fig. 2 , we indeed find a re-entrant superfluid at particle densities for which < R o . Intermediate densities A distinctive consequence of the soft-core interaction is that the energy cost for forming close particle pairs is bound by V 0 . This potentially enables the formation of crystalline phases with N > N s above a critical density where doubly occupied lattice sites become energetically favourable on increasing the lattice constant. As expected for a triangular crystal, the lattice constant decreases as a =( ρ /2) −1/2 at small densities. However, around a ≈1.4 R c it increases again and settles to a density-independent value of a 0 ≃ 1.6 R c on further increase of ρ . The corresponding volume of the unit cell A = provides a measure of the lattice occupancy N / N s = Aρ , which is also shown in Fig. 2 . The transition to cluster crystals occurs at Aρ ≈1.5. This indeed coincides with the critical density for crystallization of the re-entrant superfluid phase. Around this density, a thin region of phase separation is found to lay in between the cluster crystal and the superfluid phase. 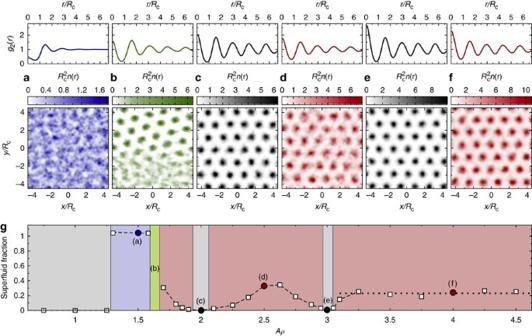Figure 3: Characterization of the different phases across the phase diagram. Panelsa–fshow the radial pair correlation functiong2(r) and the particle density distributionn(r) (see Methods section) forρU=32 and different values ofAρ, indicated ing. Panelgdisplays the superfluid fractionfsas a function ofAρ, covering all phases indicated inFig. 2. Global superfluidity is not well defined in the phase-separation region (green area) and therefore omitted. The horizontal dotted line shows theρ→∞ limit offsfor a density-wave supersolid, obtained from a mean-field evaluation following the approach of Leggett58. Figure 3b shows a typical example for the particle density distribution in this region. Two distinct coexisting phases can be recognized: a crystal phase with exactly two particles per site (upper part of the figure) and a superfluid phase (lower part). We have carefully checked that the occurrence of this phase-separated state is not an artifact of the simulations by performing accurate annealing and by choosing different initial conditions, such as random and different crystalline configurations. Figure 3: Characterization of the different phases across the phase diagram. Panels a – f show the radial pair correlation function g 2 ( r ) and the particle density distribution n ( r ) (see Methods section) for ρ U =32 and different values of Aρ , indicated in g . Panel g displays the superfluid fraction f s as a function of Aρ , covering all phases indicated in Fig. 2 . Global superfluidity is not well defined in the phase-separation region (green area) and therefore omitted. The horizontal dotted line shows the ρ →∞ limit of f s for a density-wave supersolid, obtained from a mean-field evaluation following the approach of Leggett [58] . Full size image Above incommensurate lattice occupations N / N s ≳ 1.5, the direct liquid–solid quantum phase transition is replaced by a first-order transition from a superfluid to a supersolid phase. The supersolid phase is approximately found to occur between the two hyperbola defined by ρU = α , with α ≈28 and α ≈38, respectively (see dotted lines in Fig. 2 ). These two lines are derived from the weak interaction limit ( U →0 and ρ →∞ with α =const. ), where mean-field theory predicts a transition to a density-wave supersolid that is determined only by the value of α (ref. 28 ). While this mean-field prediction becomes exact in the high-density limit (see Fig. 2 ), the situation is dramatically different at moderate densities where the discrete nature of the particles plays a significant role. This gives rise to the emergence of supersolid regions with a lobe structure, which vanish at commensurate lattice occupations N / N s =2 and N / N s =3. There, we find a direct transition between a superfluid and an insulating solid phase. This behaviour is illustrated in Fig. 3 where the superfluid fraction, f s , is shown as a function of Aρ for α =32, that is, in between the two dotted lines in Fig. 2 . As shown in Fig. 3c,e , at Aρ =2 and Aρ =3 one finds a commensurate crystal with exactly N / N s =2 ( Fig. 3c ) and N / N s =3 ( Fig. 3e ) particles per lattice site, respectively, and vanishing superfluidity ( Fig. 3g ). Importantly, the crystal structure in between these two densities is practically unchanged, as seen by comparing the particle density distributions n ( r ) and density–density correlation functions g 2 ( r ) in Fig. 3c–e . However, the incommensurate lattice filling N / N s and the resulting fluctuations of individual site occupations enables particles to tunnel between the sites. This gives rise to a non-vanishing superfluid fraction of the crystal, which can assume sizable values of f s =0.3 for N / N s ≈ Aρ =2.5. High densities For higher densities Aρ >3, the scenario described above changes considerably. As shown in Fig. 3g , the superfluid fraction approaches a constant, density-independent value f s ≈0.24 with increasing ρ . In particular, for an average commensurate filling N / N s =4 there is no direct phase transition between a superfluid and a solid insulating phase, and instead the supersolid phase persists with no significant difference to the case of incommensurate lattice occupancies N / N s ≠4. This behaviour signals a crossover to the regime where the supersolid phase can be understood in terms of a density-modulated superfluid [2] , [26] , [27] , [28] , [39] , where the discrete nature of the particles becomes irrelevant. In this limit, the superfluid–supersolid quantum phase transition is well captured by a mean-field description [26] , [28] , [40] . It predicts a transition point at α = ρU =28.2 as well as a superfluid fraction that is solely determined by the value α , and yields f s =0.23 for α =32. As shown in Figs 2 and 3g , both predictions are well confirmed by our Monte Carlo results for Aρ ≳ 3.5, suggesting that the transition to density-wave supersolidity takes place at a surprisingly small number of only N / N s ≈3.5 particles per lattice site. Defect delocalization The most interesting behaviour takes place around the superfluid–solid quantum phase transition at N / N s =2. 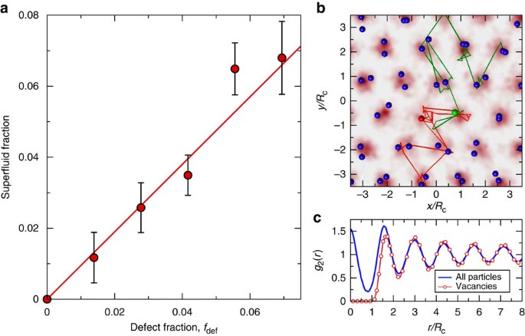Figure 4: Defect-induced superfluidity. Panelashows the superfluid fraction in a doubly occupied solid (N/Ns=2) as a function of the fraction of defects in the form of singly occupied sites for fixedU=31 and varying particle number betweenN=139 and 144. ForN=144, the system forms an insulating commensurate solid withNs=72 doubly occupied sites. Decreasing the particle number does not affectNsbut leads to the formation of a small fractionfdef=(2Ns−N)/Nsof singly occupied lattice sites. Panelbshows the particle density (colour code) forfdef=0.03, obtained from a Monte Carlo configuration along with the particle positions (spheres) for a single imaginary time slice. The two initially adjacent vacancies (red and green sphere) delocalize, as indicated by the corresponding imaginary time trajectories. Accordingly, the vacancy–vacancy pair correlation function (red), shown incforfdef=0.07, resembles theg2(r) of the underlying crystal (blue), as expected for a delocalized, very dilute gas of repulsive bosons. The error bars in panelarepresent statistical uncertainties of the Monte Carlo sampling. Figure 4 provides a more detailed look at the transition between the insulating crystal and the supersolid phase, that is, for U =31 and N / N s ≈2. Starting from the insulating solid with doubly occupied lattice sites, we successively remove a small number of particles from randomly chosen sites and monitor the superfluid fraction of the resulting new ground state obtained from our simulations. Removing a small number of particles does not cause structural changes of the ground state but rather creates a small fraction f def =(2 N s − N )/ N s of zero-point crystal defects in the form of singly occupied sites. An analysis of the Monte Carlo configurations shows that defects do not cluster and instead delocalize, as illustrated in Fig. 4b . This is also confirmed by the vacancy–vacancy pair correlation function, as shown in Fig. 4c . For r ≳ a 0 , it closely resembles the g 2 ( r ) of the underlying solid, as expected for a very dilute gas of repulsive bosons. Indeed, we find a finite superfluid fraction even for small defect concentrations, which increases linearly with f def . We have verified that this finding is pertinent to the ground state and not to a metastable configuration by performing simulations with different initial conditions, including clustered defects. The observed behaviour is, thus, consistent with defect-induced supersolidity according to the ALC scenario, and constitutes the central result of this work. Figure 4: Defect-induced superfluidity. Panel a shows the superfluid fraction in a doubly occupied solid ( N / N s =2) as a function of the fraction of defects in the form of singly occupied sites for fixed U =31 and varying particle number between N =139 and 144. For N =144, the system forms an insulating commensurate solid with N s =72 doubly occupied sites. Decreasing the particle number does not affect N s but leads to the formation of a small fraction f def =(2 N s − N )/ N s of singly occupied lattice sites. Panel b shows the particle density (colour code) for f def =0.03, obtained from a Monte Carlo configuration along with the particle positions (spheres) for a single imaginary time slice. The two initially adjacent vacancies (red and green sphere) delocalize, as indicated by the corresponding imaginary time trajectories. Accordingly, the vacancy–vacancy pair correlation function (red), shown in c for f def =0.07, resembles the g 2 ( r ) of the underlying crystal (blue), as expected for a delocalized, very dilute gas of repulsive bosons. The error bars in panel a represent statistical uncertainties of the Monte Carlo sampling. Full size image Supersolidity in this system is the consequence of two unique features of soft-core bosons. First, the energy cost for forming close particle pairs is bound by V 0 , which facilitates the formation of cluster crystals that naturally entail zero-point defects. Second, the dynamics and interaction of these defects differs fundamentally from those of conventional solids. In the latter case, vacancies and interstitials induce displacement fields that lead to purely attractive defect interactions [21] , [23] , [24] , [44] and, therfore, prevent a delocalization of defects [21] . In cluster solids, on the other hand, defect interactions are purely repulsive, since they interact via the same underlying particle interaction V ( r ) of equation (1). In the present case, the transition between these two regimes is controlled by the particle density. For Aρ ≳ 1.5 delocalized zero-point defects allow for the formation of supersolid phases. Below this density particles do not explore the soft-core part of the interaction potential, such that defects are attractive and supersolidity is absent consistent with the results of Boninsegni et al. [21] Around the transition region Aρ ≈1.5 neither picture applies, and one observes separation between a superfluid and a doubly occupied, insulating cluster solid. Preliminary calculations based on path-integral Langevin dynamics [45] suggest that in this region structural and dynamical heterogeneity can give rise to a quantum glass phase at finite temperature. Having identified a physical system that facilitates defect-induced supersolidity, we hope that this work will provide useful guidance for future experiments and initiate further theoretical explorations. An important question concerns the general features of the interaction potential that are required to maintain the type of supersolid states described in this work. While the emergence of weakly interacting density-wave supersolids is largely insensitive to the detailed shape of the soft-core interaction, the low-density physics described in this work may be strongly affected. In fact, it seems reasonable to expect an interesting competition between intra- and inter-site interactions within the self-assembled crystal that will depend on the long-range tail of the particle interactions. Moreover, the role of the dimensionality and confined geometries of finite systems represent another outstanding issue, and in particular their role for frustration effects with regard to defect delocalization. While the considered interactions do not straightforwardly occur in natural crystals, they can be designed in ultracold atom experiments. Recent experiments with Bose–Einstein condensates in optical cavities have already demonstrated a density-wave supersolid due to the breaking of a discrete translational symmetry [46] , [47] and theoretical work has devised several schemes [30] , [31] for the manipulation of long-range interactions between polar molecules by external fields. Moreover, far off-resonant excitation of high lying Rydberg states [28] , [29] , [48] in degenerate atomic gases [49] , [50] , [51] was shown to realize interactions of the type of equation (1). Following Maucher et al. [29] , such a Rydberg dressing of 87 Rb condensates to Rb(35 p 3/2 ) states [52] with a laser detuning of ~500 MHz, and an intensity of 100 kW cm −2 would produce a sizeable interaction strength of U ~35. While we have focussed here on the zero-temperature limit, we have also performed finite-temperature simulations, showing that these parameters will permit the experimental observation of defect-induced supersolid phases for temperatures T ≲ 10 nK, around typical densities ~10 8 cm −2 and with a condensate lifetime of ~30 ms, limited by radiative decay of the weakly admixed Rydberg state. Recent experimental breakthroughs reporting the first observation of Rydberg interaction effects in a laser-driven Bose–Einstein condensate [53] hold high promise for the prospective realization of the setting described in this work. Numerical details Our numerical results were obtained from path-integral Monte Carlo simulations [54] based on the continuous-space worm algorithm [55] to determine the equilibrium properties of equation (2) in the canonical ensemble, that is, at a fixed temperature T and a fixed particle number, chosen between N =100 and 400. From these simulations we obtain, for example, density profiles, n ( r )=‹ ( r − r i ( t ))› t , and pair correlation functions, g 2 ( r )=[2π n ( N −1) r ] −1 ‹ ( r − r ij ( t ))› t , as well as the superfluid fraction f s , computed from the area estimator, as described in Sindzingre et al. [56] and Pollock et al. [57] Here r ij =| r j − r i |, r i are the positions of the i =1,…, N particles, and ‹..› t denotes an average of the corresponding imaginary time trajectories r i ( t ). The properties of the system ground state were obtained by extrapolating to the limit of zero temperature, that is, by lowering the temperature until observables, such as the total energy, superfluid fraction and pair correlations did not change on further decrease of T . Moreover, the size of our two-dimensional simulation box with periodic boundary conditions was varied to assure insensitivity to system size. The calculated observables were used to construct the phase diagram. The first-order superfluid–normal solid transition is detected by an abrupt increase of the maximum value ( S max ) of the static structure factor S ( k )=1+ ρ ∫d r e i kr ( g 2 ( r )−1) and a simultaneous vanishing of the superfluid fraction. The superfluid–supersolid transition is characterized by a jump of S max and an abrupt decrease of the superfluid fraction from f s ≈1 to a finite value f s >0, while the supersolid–normal solid transition is signalled by the vanishing of f s . How to cite this article: Cinti, F. et al. Defect-induced supersolidity with soft-core bosons. Nat. Commun. 5:3235 doi: 10.1038/ncomms4235 (2014).